Metabolite-sensing receptors GPR43 and GPR109A facilitate dietary fibre-induced gut homeostasis through regulation of the inflammasome Diet and the gut microbiota may underpin numerous human diseases. A major metabolic product of commensal bacteria are short-chain fatty acids (SCFAs) that derive from fermentation of dietary fibre. Here we show that diets deficient or low in fibre exacerbate colitis development, while very high intake of dietary fibre or the SCFA acetate protects against colitis. SCFAs binding to the ‘metabolite-sensing’ receptors GPR43 and GPR109A in non-haematopoietic cells mediate these protective effects. The inflammasome pathway has hitherto been reported as a principal pathway promoting gut epithelial integrity. SCFAs binding to GPR43 on colonic epithelial cells stimulates K + efflux and hyperpolarization, which lead to NLRP3 inflammasome activation. Dietary fibre also shapes gut bacterial ecology, resulting in bacterial species that are more effective for inflammasome activation. SCFAs and metabolite receptors thus explain health benefits of dietary fibre, and how metabolite signals feed through to a major pathway for gut homeostasis. The basis of numerous human diseases may relate to diet and the actions of gut microbes and their metabolites [1] , [2] , [3] , [4] . For the most part, this has been studied in mice or humans that have been fed a high-fat diet [5] , [6] or that regularly consume a Western diet [3] , [7] ; however another proposal is that it is low consumption of dietary fibre that may negatively impact on health [4] , [8] . Dietary fibre has been promoted for its health benefits, and high-fibre consumption has been reported as beneficial in numerous diseases including inflammatory bowel diseases [9] , [10] . While the recommended consumption of fibre in the United States of America is 38 g per day for men, the real consumption is less than half of this, with an average of ~15 g (ref. 9 ). This low consumption may underlie many ‘Western lifestyle’ diseases, and low consumption of dietary fibre in humans correlates with increased mortality due to various conditions [11] . However, while dietary fibre is considered beneficial for gut health, and health in general [9] , the mechanisms behind the actions of fibre are still poorly understood. Dietary fibre is fermented to short-chain fatty acids (SCFAs) in the gastrointestinal (GI) tract through the actions of commensal anaerobic bacteria. The SCFAs produced in the gut are mainly acetate, butyrate and propionate, with acetate being released in highest quantities and distributed systemically through the blood. SCFAs can modulate cell functions either by inhibiting histone deacetylase activity, and thereby affecting gene transcription, or through the activation of ‘metabolite-sensing’ G-protein coupled receptors (GPCRs) such as GPR43 (ref. 12 ). We have demonstrated previously that GPR43-deficient mice show exacerbated or unresolving inflammation in models such as dextran sulphate sodium (DSS)-induced colitis [12] . However, whether the beneficial effects of dietary fibre on DSS colitis involve GPR43 remains uncertain. Acetate and propionate are the main SCFAs that bind GPR43 (reviewed in ref. 13 ). Acetate is known to promote gut epithelial integrity through undefined mechanisms [14] . Currently, the inflammasome pathway and production of the cytokine interleukin (IL)-18 are the best-characterized molecular mechanisms for maintenance of epithelial integrity, repair and intestinal homeostasis [15] , [16] , [17] , [18] , [19] . Factors that trigger activation of the inflammasome in gut epithelium are poorly understood. Regardless, its assembly results in the cleavage of the enzyme caspase 1 into its active form, which then cleaves pro-IL-18 into IL-18. IL-18 is a cytokine that promotes gut epithelial integrity [15] . Mice deficient in the NLRP3 or NLRP6 inflammasome components develop exacerbated colitis in the DSS model, at least in most studies [15] , [17] . Likewise mice deficient in caspase 1 or IL-18 show exacerbated colitis [15] . Thus, two separate and seemingly unrelated fields have been implicated in gut homeostasis—dietary fibre and acetate on the one hand, and the inflammasome pathway and IL-18 on the other. In the present work, we aimed to uncover mechanisms whereby dietary fibre produces health benefits, particularly in the gut. We fed mice diets either deficient, low or enriched in fibre (designed based on the Dietary Reference Intake (DRI) of 14 g per 1,000 kcal) and then treated mice with DSS to induce intestinal damage and colitis. We found that the degree of colitis was inversely proportional to the amount of fibre in the diet. We used Gpr43 −/− , Gpr109a −/− , Nlrp3 −/− and Nlrp6 −/− mice, as well as bone marrow chimaera models, to show that the beneficial effects of a high-fibre diet involved the activation of GPR43 and GPR109A in the gut epithelium, and downstream activation of the NLRP3 inflammasome pathway. Finally, we found that K + efflux could trigger inflammasome activation in vitro , and that SCFAs could activate the inflammasome in these cells through a mechanism that involves GPCR-mediated hyperpolarization secondary to Ca 2+ mobilization. Dietary fibre also altered gut microbial ecology to yield a microbiome that was highly efficient in activating the epithelial inflammasome pathway and stimulating IL-18 production. Thus, dietary fibre, gut microbiota and downstream pathways involving GPR43, GPR109A and the inflammasome combine to promote gut homeostasis. Low-fibre diets aggravate DSS colitis while high-fibre protects While high amounts of dietary fibre is known to be beneficial for gut health, very few studies have investigated the impact of diets deficient or low in fibre. To achieve this, we fed mice on diets deprived, reduced or enriched in fibre. We designed our diets based on the DRI that recommends an intake of fibre of 14 g per 1,000 kcal consumed in humans ( www.nih.gov ). The daily food intake of mice fed on our high-fibre diet (35% crude fibre) was 7.45 g food per day per mouse, which represents a consumption of 136 g per 1,000 kcal, which is equivalent to 9.7 times more than the recommended amount of fibre. Mice fed on low-fibre diet (2.3% fibre) consumed 6.3 g food per day per mouse, representing a consumption of fibre of 5.1 g per 1,000 kcal, which is 2.7 times less than the recommended amount, equivalent to typical consumption in Western countries. Mice were fed on zero-, low- or high-fibre diets and assessed in the DSS model of colitis, which involves intestinal injury, inflammation and tissue repair [20] . DSS colitis in mice is characterized by the development of diarrhoea and colonic inflammation leading to blood in the faeces, measured by a clinical score, destruction of colonic tissue assessed by histological scoring of colonic tissue, as well as colon shortening. When compared with mice fed on a diet deficient in fibre, high-fibre (or normal chow; Supplementary Fig. 1 ) feeding protected from DSS colitis with a significantly improved clinical score ( Fig. 1a ), reduced weight loss ( Fig. 1b ) and increased colon length ( Fig. 1c ). This was confirmed by the fact that mice fed on resistant starch, which also increases SCFA levels, were protected from DSS-induced colitis ( Supplementary Fig. 2 ). Consumption of a more physiological diet with a reduced amount of fibre had similar deleterious effects with worse DSS colitis development as shown by increased clinical scores, decreased colon length and worse tissue damage ( Fig. 1d–g ) when compared with high-fibre-fed mice. Interestingly, zero-fibre-fed mice developed worse disease than low-fibre-fed mice ( Fig. 1d–g ), suggesting that fibre has a dose effect on disease development. The high-fibre diet yielded very high levels of acetate in serum of mice, ~200 μM ( Fig. 1h ) and in faeces ( Fig. 1i ) compared with mice fed on zero-fibre diet. To determine whether changes in acetate levels might account for protection or increased susceptibility to develop DSS colitis, specific-pathogen-free mice received different doses of acetate in drinking water for 3 weeks before treatment with DSS. While neither 100 nor 200 mM acetate were protective in SPF mice, we found that 300 mM acetate significantly improved clinical scores ( Fig. 1j ) and tissue inflammation ( Fig. 1k ). Thus, deficiency of dietary fibre aggravated development of DSS colitis, while high consumption of dietary fibre or treatment with acetate had protective effects. 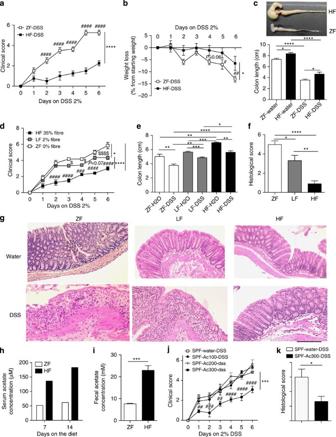Figure 1: Fibre and acetate protect from DSS-induced colitis. (a–c) Clinical score (a), weight loss (b) and colon length (c) assessed on female mice treated with 2% DSS for 6 days after being fed on either zero-fibre (ZF-DSS) or high-fibre (HF-DSS) diets for a week prior and during DSS treatment (n=6 mice per group repeated three times). (d–f) Clinical score (d), colon length (e), histological score assessed on female mice treated or not with 2% DSS for 6 days after being fed on either ZF, low-fibre (LF) and on HF diets (f) for a week prior and during DSS treatment (n=6 mice minimum per group repeated twice). (g) Representative haematoxylin and eosin-stained colonic sections. (h,i) Serum acetate levels fromn=6 female mice fed for 7 or 14 days (h) and faecal acetate from mice fed on diets for 14 days (i). (j) Clinical score assessed on mice treated for 3 weeks before 6 days on DSS treatment with 100, 200 and 300 mM acetate or water (n=6 mice per group repeated twice). (k) Histological score assessed on colonic section of mice treated with 300 mM acetate or water before DSS; scale bar, 200 μm. The results are shown as mean±s.e.m. ofn=5 mice minimum per group. With *P<0.05, ***P<0.001 and ****P<0.0001 determined as group effect by two-way analysis of variance,####P<0.001 determined by Bonferroni’s multiple analysis (a),P=0.07,$P<0.05 and
    
P<0.0001 comparing ZF and LF; and###P<0.001 and####P<0.0001 comparing HF and LF (d),##P<0.01,###P<0.001 and####P<0.0001 comparing 300 mM acetate with water groups (j) by Tukey’s multiple comparison analysis,P=0.06,#P<0.05,##P<0.01, *P<0.05, **P<0.01 and ****P<0.001 byt-test. Figure 1: Fibre and acetate protect from DSS-induced colitis. ( a – c ) Clinical score ( a ), weight loss ( b ) and colon length ( c ) assessed on female mice treated with 2% DSS for 6 days after being fed on either zero-fibre (ZF-DSS) or high-fibre (HF-DSS) diets for a week prior and during DSS treatment ( n =6 mice per group repeated three times). ( d – f ) Clinical score ( d ), colon length ( e ), histological score assessed on female mice treated or not with 2% DSS for 6 days after being fed on either ZF, low-fibre (LF) and on HF diets ( f ) for a week prior and during DSS treatment ( n =6 mice minimum per group repeated twice). ( g ) Representative haematoxylin and eosin-stained colonic sections. ( h , i ) Serum acetate levels from n =6 female mice fed for 7 or 14 days ( h ) and faecal acetate from mice fed on diets for 14 days ( i ). ( j ) Clinical score assessed on mice treated for 3 weeks before 6 days on DSS treatment with 100, 200 and 300 mM acetate or water ( n =6 mice per group repeated twice). ( k ) Histological score assessed on colonic section of mice treated with 300 mM acetate or water before DSS; scale bar, 200 μm. The results are shown as mean±s.e.m. of n =5 mice minimum per group. With * P <0.05, *** P <0.001 and **** P <0.0001 determined as group effect by two-way analysis of variance, #### P <0.001 determined by Bonferroni’s multiple analysis ( a ), P =0.07, $ P <0.05 and 
    
 P <0.0001 comparing ZF and LF; and ### P <0.001 and #### P <0.0001 comparing HF and LF ( d ), ## P <0.01, ### P <0.001 and #### P <0.0001 comparing 300 mM acetate with water groups ( j ) by Tukey’s multiple comparison analysis, P =0.06, # P <0.05, ## P <0.01, * P <0.05, ** P <0.01 and **** P <0.001 by t -test. Full size image Dietary fibre protects from DSS colitis via GPR43 and GPR109A SCFAs such as acetate promote gut epithelial integrity [14] , [21] . An indication as to the molecular pathways used by SCFAs was suggested through the use of inhibitors of GPCR signalling [21] . We therefore determined whether the beneficial effects of fibre on DSS colitis were mediated via the metabolite-sensing GPCRs GPR43 (also referred to as FFA2) and GPR109A (also referred to as HCA2). Wild-type (WT) mice fed a high-fibre diet, as opposed to a zero-fibre diet, showed improved clinical scores from early stages of the DSS model ( Fig. 2a ), whereas Gpr43 −/− mice on a high-fibre diet showed only a slight improvement in clinical scores ( P <0.05, group effect by analysis of variance; Fig. 2a ). In Gpr43 −/− mice, the high-fibre diet failed to reduce weight loss ( Supplementary Fig. 3a ) to improve colon length ( Fig. 2b ) or to reduce damage to colonic tissue ( Fig. 2c and Supplementary Fig. 3b ). Because GPR43 did not account for 100% of the beneficial effects of a high-fibre diet, at least by clinical score, we next tested GPR109A, a receptor expressed by colonic epithelial cells [22] that binds the SCFA butyrate and the fatty acid-derived ketone body (D)-beta-hydroxybutyrate [23] . We found that protection in the DSS model provided by high-fibre diet was GPR109A dependent, at least by clinical scores ( Fig. 2d ) and histology scores ( Fig. 2e and Supplementary Fig. 3d ), but less so by colon length ( Fig. 2f ). We next determined the contribution of immune versus non-immune cells to the protection provided by high-fibre feeding on DSS colitis using bone marrow chimaeras. After 8 weeks of bone marrow reconstitution, diets were started and DSS colitis induced by DSS in the drinking water. High-fibre-fed mice deficient for GPR43 in the haematopoietic compartment (irradiated C57BL6 mice reconstituted with Gpr43 −/− bone marrow cells) showed similar clinical scores, colon lengths and histological scores ( Supplementary Fig. 4a–c and Fig. 2g,h ) as control mice (irradiated C57BL6 mice reconstituted with C57BL6 bone marrow). In contrast, we found that the beneficial role of high-fibre feeding relied predominantly on GPR43 expression by non-haematopoietic cells ( Fig. 2g,h ) when compared with high-fibre-fed control mice. Altogether, these data show that beneficial effects of dietary fibre are mediated through effects on GPR43 within the non-haematopoeitic compartment, probably the gut epithelium. Similarly, absence of GPR109A in the non-haematopoeitic compartment abrogated the protective effects of fibre in DSS colitis ( Supplementary Fig. 5 ), presumably in the epithelium, a site of GPR109A expression [22] . 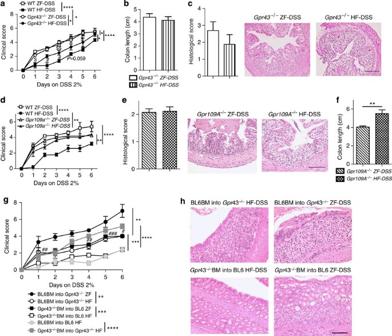Figure 2: Beneficial effects of fibre in DSS colitis are mediated through GPR43 and GPR109A, and expressed in non-haematopoietic cells. Clinical scores measured in WT (a,d), inGpr43−/−mice (a) and inGpr109A−/−mice (d) fed on zero-fibre (ZF) or on high-fibre (HF) diets for 7 days prior and during the 6 days treatment with 2% DSS. (b,f) Colon length measured at day 6 in DSS-treatedGpr43−/−mice (b) orGpr109A−/−mice (f) versus WT mice fed on ZF or HF diets. (c,e) Histological score and representative haematoxylin and eosin (H&E)-stained colonic sections of HF-DSS- and ZF-DSS-fedGpr43−/−(c) orGpr109A−/−(e) mice treated with DSS (n=6 mice per group, repeated twice); scale bars, 200 μm. (g) Clinical scores assessed in irradiatedGpr43−/−mice reconstituted withGpr43−/−bone marrow (BM;Gpr43−/−BM intoGpr43−/−) fed on HF diet (n=6) or with WT BM (BL6BM intoGpr43−/−) fed on HF (n=5) or on ZF (n=5) diets, in irradiated WT mice reconstituted with WT BM cells (BL6BM into BL6) fed on HF diet (n=5) or in irradiated WT mice reconstituted withGpr43−/−BM (Gpr43−/−BM into BL6) fed on HF (n=10) or on ZF (n=10) diets. Mice were fed on diets for a week prior and during treatment with 2% DSS for 6 days. (h) Representative H&E-stained colonic sections of HF-DSS and ZF-DSS-fed irradiated WT mice reconstituted withGpr43−/−BM cells (Gpr43−/−BM into BL6) and in irradiatedGpr43−/−mice reconstituted with WT BM cells (BL6BM intoGpr43−/−); scale bar, 200 μm. The results are shown as mean±s.e.m. of at leastn=6 mice per group repeated twice. With *P<0.05, **P<0.01, ***P<0.001 and ****P<0.0001 as group effect as determined by two-way analysis of variance,#P<0.05 as comparison between WT HF-DSS andGpr43−/−HF-DSS,$P<0.05,$$P<0.01 as differences betweenGpr43−/−HF-DSS versus ZF-DSS determined by Tukey’s multiple analysis (a),#P<0.05,##P<0.01,####P<0.0001 as comparison between WT HF-DSS andGpr109A−/−HF-DSS by Sidak’s multiple comparison analysis (d),#P<0.05,##P<0.01 and###P<0.001 as comparison between BL6BM intoGpr43−/−HF versus BL6BM into BL6 HF determined by Tukey’s multiple comparison analysis (g) and **P<0.01 byt-test. Figure 2: Beneficial effects of fibre in DSS colitis are mediated through GPR43 and GPR109A, and expressed in non-haematopoietic cells. Clinical scores measured in WT ( a , d ), in Gpr43 −/− mice ( a ) and in Gpr109A −/− mice ( d ) fed on zero-fibre (ZF) or on high-fibre (HF) diets for 7 days prior and during the 6 days treatment with 2% DSS. ( b , f ) Colon length measured at day 6 in DSS-treated Gpr43 −/− mice ( b ) or Gpr109A −/− mice ( f ) versus WT mice fed on ZF or HF diets. ( c , e ) Histological score and representative haematoxylin and eosin (H&E)-stained colonic sections of HF-DSS- and ZF-DSS-fed Gpr43 −/− ( c ) or Gpr109A −/− ( e ) mice treated with DSS ( n =6 mice per group, repeated twice); scale bars, 200 μm. ( g ) Clinical scores assessed in irradiated Gpr43 −/− mice reconstituted with Gpr43 −/− bone marrow (BM; Gpr43 −/− BM into Gpr43 −/− ) fed on HF diet ( n =6) or with WT BM (BL6BM into Gpr43 −/− ) fed on HF ( n =5) or on ZF ( n =5) diets, in irradiated WT mice reconstituted with WT BM cells (BL6BM into BL6) fed on HF diet ( n =5) or in irradiated WT mice reconstituted with Gpr43 −/− BM ( Gpr43 −/− BM into BL6) fed on HF ( n =10) or on ZF ( n =10) diets. Mice were fed on diets for a week prior and during treatment with 2% DSS for 6 days. ( h ) Representative H&E-stained colonic sections of HF-DSS and ZF-DSS-fed irradiated WT mice reconstituted with Gpr43 −/− BM cells ( Gpr43 −/− BM into BL6) and in irradiated Gpr43 −/− mice reconstituted with WT BM cells (BL6BM into Gpr43 −/− ); scale bar, 200 μm. The results are shown as mean±s.e.m. of at least n =6 mice per group repeated twice. With * P <0.05, ** P <0.01, *** P <0.001 and **** P <0.0001 as group effect as determined by two-way analysis of variance, # P <0.05 as comparison between WT HF-DSS and Gpr43 −/− HF-DSS, $ P <0.05, 
    P <0.01 as differences between Gpr43 −/− HF-DSS versus ZF-DSS determined by Tukey’s multiple analysis ( a ), # P <0.05, ## P <0.01, #### P <0.0001 as comparison between WT HF-DSS and Gpr109A −/− HF-DSS by Sidak’s multiple comparison analysis ( d ), # P <0.05, ## P <0.01 and ### P <0.001 as comparison between BL6BM into Gpr43 −/− HF versus BL6BM into BL6 HF determined by Tukey’s multiple comparison analysis ( g ) and ** P <0.01 by t -test. Full size image Dietary fibre and SCFAs facilitate inflammasome activation Currently, the inflammasome pathway and production of the cytokine IL-18 are the best-characterized molecular mechanisms for maintenance of epithelial integrity, repair and intestinal homeostasis [15] , [16] , [17] , [18] . Since dietary fibre as well as SCFAs are known contributors to epithelial integrity [14] , [21] , [24] , we examined the influence of diet and the SCFA receptors GPR43 on inflammasome activation and IL-18 production. Western blots of colonic epithelial cells following DSS colitis showed that zero-fibre feeding yielded very low to absent levels of the cleaved form of caspase 1 ( Fig. 3a ) and of IL-18 ( Fig. 3b ), in contrast to high-fibre feeding. High-fibre diet resulted in increased levels of IL-18 in serum, even before induction of DSS colitis, and this was markedly enhanced following DSS induction, and was dependent on GPR43 ( Fig. 3c ) and on GPR109A ( Fig. 3d ). High-fibre feeding did not affect expression of IL-1β, a cytokine considered redundant with respect to the protective effects of the inflammasome pathway in DSS colitis [15] , [16] . Interestingly, we found that IL-18 was increased under basal conditions not only under high-fibre-feeding conditions ( Fig. 3c,d ) but also in SPF mice treated with 200 and 300 mM acetate ( Fig. 3e ). As observed under high-fibre-feeding conditions, treatment with 300 mM acetate (that significantly alleviated DSS colitis; Fig. 1j,k ) was also associated with significantly higher serum IL-18 ( Fig. 3f ). Altogether, these results show that the beneficial effects of high-fibre feeding and acetate treatment in DSS colitis are associated with increased inflammasome activation, and this occurred in a GPR43- and GPR109A-dependent manner. 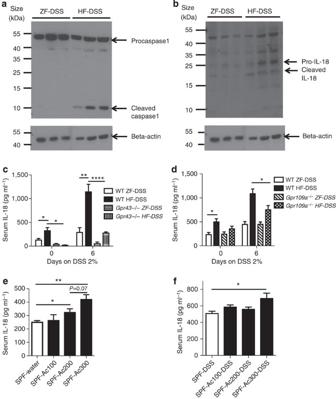Figure 3: High-fibre diet and acetate facilitates inflammasome activation in colonic epithelial cells through GPR43. (a,b) Measurement by western blot of caspase 1 (a) and of IL-18 (b) on protein extracted from colonic intestinal epithelial cells from mice fed on zero-fibre (ZF) versus high-fibre (HF) diet fed for 7 days prior and during 6 days treatment with 2% DSS. Each column represents one mouse. The experiment has been repeated three times. (c–e) IL-18 measured by enzyme-linked immunosorbent assay on serum isolated from WT and fromGpr43−/−mice fed on ZF or HF (n=5 mice in WT groups andn=6 mice inGpr43−/−groups, repeated twice) (c) and from WT and fromGpr109A−/−mice fed on ZF or HF (n=5 mice in WT groups andn=5 mice inGpr109A−/−groups, repeated twice) (d) at days 0 and 6 of treatment on DSS, (c) on serum isolated from mice treated for 3 weeks on 100, 200 and 300 mM acetate (e) then treated for 6 days on DSS (n=6 mice per group) (f). The results are shown as mean±s.e.m. WithP=0.07, *P<0.05, **P<0.01, ****P<0.0001 byt-test. Figure 3: High-fibre diet and acetate facilitates inflammasome activation in colonic epithelial cells through GPR43. ( a , b ) Measurement by western blot of caspase 1 ( a ) and of IL-18 ( b ) on protein extracted from colonic intestinal epithelial cells from mice fed on zero-fibre (ZF) versus high-fibre (HF) diet fed for 7 days prior and during 6 days treatment with 2
$ P <0.001 and 
    
 P <0.0001 comparing Nlrp3 −/− ZF versus HF and ### P <0.001 and #### P <0.0001 comparing Nlrp3 −/− HF versus WT HF by Bonferroni’s multiple comparison analysis ( a ), ### P <0.001 and #### P <0.0001 comparing Nlrp6 −/− HF versus ZF determined by Tukey’s multiple comparison analysis ( e ), and with P =0.05, ** P <0.01, *** P <0.001 and **** P <0.0001 as determined by t -test. NS, not significant. Full size image Fibre protects through NLRP3 in non-haematopoietic cells To determine in which compartment expression of NLRP3 was required to mediate the beneficial effects of fibre, we used bone marrow chimaeras. Mice lacking NLRP3 expression specifically in the non-immune compartment showed little beneficial effect of high-fibre diet on clinical scores, colon length and histological scores when compared with mice lacking NLRP3 in the haematopoietic compartment ( Fig. 5a–d ). 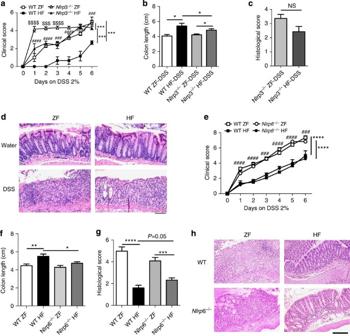Figure 4: Fibre mediates its beneficial effects on DSS colitis by activating the NLRP3 but not NLRP6 inflammasome. Clinical scores measured in WT (a,e), inNlrp3−/−mice (a) (n=6 mice per group exceptNlrp3−/−HFn=5, experiment done twice) and inNlrp6−/−(n=6 mice per group) (e) mice fed on zero-fibre (ZF) or on high-fibre (HF) diets and treated for 6 days with 2% DSS. (b,f) Colon length, (d,h) histological score and representative haematoxylin and eosin-stained colonic sections of WT,Nlrp3−/−mice (b–d) and inNlrp6−/−(f–h) fed in ZF or HF before DSS treatment; scale bars, 200 μm. The results are shown as mean±s.e.m.. With ***P<0.001 and ****P<0.0001 as determined by analysis of variance as group effect,
    P<0.001 and
$$P<0.0001 comparingNlrp3−/−ZF versus HF and###P<0.001 and####P<0.0001 comparing Nlrp3−/−HF versus WT HF by Bonferroni’s multiple comparison analysis (a),###P<0.001 and####P<0.0001 comparingNlrp6−/−HF versus ZF determined by Tukey’s multiple comparison analysis (e), and withP=0.05, **P<0.01, ***P<0.001 and ****P<0.0001 as determined byt-test. NS, not significant. Thus high-fibre diet mediates its protective effects, at least in part, through NLRP3 activation, most likely within the colonic epithelium. 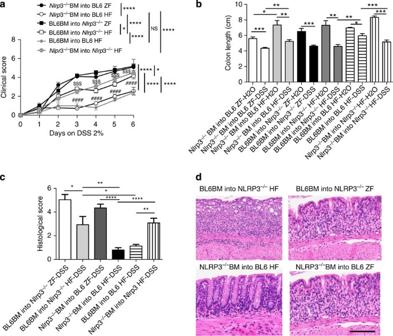Figure 5: Expression of NLRP3 in non-haematopoietic cells is necessary for the beneficial effects of high-fibre feeding in DSS colitis. Clinical score (a), colon length (b), histological score (c) and representative haematoxylin and eosin-stained colonic sections (d) were determined in irradiated WT mice reconstituted withNlrp3−/−bone marrow (BM) cells (Nlrp3−/−BM into BL6) fed on zero fibre (ZF;n=9) and on high-fibre diet (HF;n=9), in irradiatedNlrp3−/−mice reconstituted with WT BM cells (BL6BM intoNlrp3−/−) fed on ZF (n=5) or on HF (n=5), in irradiated WT mice reconstituted with WT BM cells (BL6BM into BL6) fed on HF (n=5), and in irradiatedNlrp3−/−mice reconstituted withNlrp3−/−BM cells (Nlrp3−/−BM intoNlrp3−/−) fed on HF (n=6) before and during treatment with 2% DSS or water. The results are shown as mean±s.e.m., scale bar=200 μm. With *P<0.05 and ****P<0.0001 as interaction of group effects as determined by analysis of variance,$$$P<0.001 comparing BL6BM intoNlrp3−/−HF versus BL6BM into BL6 HF,####P<0.0001 comparingNlrp3−/−BM into BL6 HF versusNlrp3−/−BM intoNlrp3−/−HF by Tukey’s multiple comparison analysis and *P<0.05 **P<0.01, ***P<0.001 and ****P<0.0001 determined byt-test. Figure 5: Expression of NLRP3 in non-haematopoietic cells is necessary for the beneficial effects of high-fibre feeding in DSS colitis. Clinical score ( a ), colon length ( b ), histological score ( c ) and representative haematoxylin and eosin-stained colonic sections ( d ) were determined in irradiated WT mice reconstituted with Nlrp 3 −/− bone marrow (BM) cells ( Nlrp3 −/− BM into BL6) fed on zero fibre (ZF; n =9) and on high-fibre diet (HF; n =9), in irradiated Nlrp3 −/− mice reconstituted with WT BM cells (BL6BM into Nlrp3 −/− ) fed on ZF ( n =5) or on HF ( n =5), in irradiated WT mice reconstituted with WT BM cells (BL6BM into BL6) fed on HF ( n =5), and in irradiated Nlrp3 −/− mice reconstituted with Nlrp3 −/− BM cells ( Nlrp3 −/− BM into Nlrp 3 −/− ) fed on HF ( n =6) before and during treatment with 2% DSS or water. The results are shown as mean±s.e.m., scale bar=200 μm. With * P <0.05 and **** P <0.0001 as interaction of group effects as determined by analysis of variance, 
    P <0.001 comparing BL6BM into Nlrp3 −/− HF versus BL6BM into BL6 HF, #### P <0.0001 comparing Nlrp3 −/− BM into BL6 HF versus Nlrp3 −/− BM into Nlrp3 −/− HF by Tukey’s multiple comparison analysis and * P <0.05 ** P <0.01, *** P <0.001 and **** P <0.0001 determined by t -test. Full size image Inflammasome activation by GPCR signalling in epithelial cells While factors promoting NLRP3 activation are well defined in immune cells, the mechanisms remain unknown in epithelial cells. In primed macrophages, at least two signals are necessary to trigger its activation, a priming phase that promotes NLRP3 gene expression and a second signal that triggers NLRP3 activation [25] . While toll-like receptor activation and tumor necrosis factor can prime inflammasome activation in macrophages [25] , [26] , signals that prime inflammasome activation in epithelial cells are unknown. Under DSS conditions, numerous bacterial products, including TLR ligands, are increased in the GI tract [27] , and these may interact with epithelial cells and contribute to their priming and inflammasome activation. To test this, HT29 were incubated with faecal contents containing mostly bacterial extract, and this effectively primed the cells as shown by a fourfold increased in NLRP3 mRNA expression ( Fig. 6a ). Membrane hyperpolarization, especially mediated by K + efflux, triggers NLRP3 activation in primed macrophages [25] . To determine whether this process was critical in epithelial cells, we incubated primed NMC460 cells, a non-cancerous human colonic epithelial cell line, in a medium deprived in K + that, by osmotic effects, is known to promote K + efflux. As observed in immune cells, we found that K + efflux promoted inflammasome activation in NMC460 cells, as shown by increased caspase 1 ( Fig. 6b ). Addition of acetate after priming also directly activated caspase 1 activation in NMC460 ( Fig. 6b ). To determine whether acetate could directly affect ion transport through the membrane epithelium, we measured the membrane potential of NMC460 ( Fig. 6c ) and HT29 ( Fig. 6d ) incubated with 10 mM acetate, a concentration reported by us and others as effective for GPR43 signalling [12] . Interestingly, 10 mM acetate induced a profound hyperpolarization in these two different human colonic epithelial cell lines ( Fig. 6c,d ). To determine whether this hyperpolarization was GPR43 dependent, we incubated CHO cells that were either transfected, or not, with a GPR43 construct (no effective GPR43 antagonists are commercially available). Interestingly, while acetate induced a profound hyperpolarization in CHO cells transfected with GPR43, ( Fig. 6e ) it did not in untransfected cells ( Fig. 6f ), indicating that GPR43 was involved the hyperpolarization induced by acetate in epithelial cells. A rise of cytoplasmic Ca 2+ can contribute to NLRP3 activation by inducing K + efflux. As previously shown by us in neutrophils [12] , we also found that acetate increased Ca 2+ levels in colonic epithelial cells ( Fig. 6g ). To determine whether the mobilization of Ca 2+ might contribute to the hyperpolarization observed after treatment with acetate, we incubated the cells with acetate in the presence of a selective calcium chelator, BAPTA-AM, to prevent this increase. We found that BAPTA-AM abrogated the hyperpolarization mediated by acetate ( Fig. 6h ). Altogether, these results show that following priming with faecal contents, hyperpolarization due to K+ efflux or successive to Ca 2+ mobilization mediated by acetate triggers inflammasome activation in human colonic epithelial cells via GPR43. 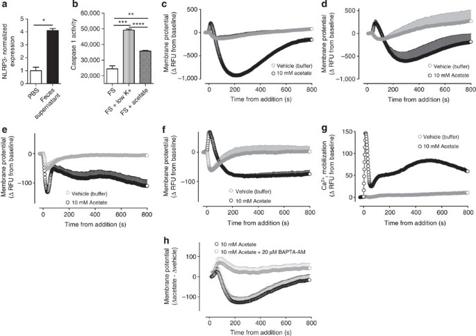Figure 6: K+efflux or hyperpolarization mediated by acetate induces inflammasome activation in primed human colonic epithelial cells. (a) NLPR3 normalized expression with GAPDH was measured in HT29 cells incubated for 2 h with diluted faecal supernatant (FS) or with PBS by real-time PCR. Results are shown as mean±s.e.m. of duplicate of a representative experiment. (b) Caspase 1 activity was measured via a fluorometric assay measuring the cleavage of the peptide YVAD-AFC. NMC460 cells were incubated with diluted FS for 4 h followed by 2 h with PBS (FS), incubated with FS for 4 h followed by 2 h in low K+medium (FS-low K+) or incubated with FS for 4 h followed by 2 h with 10 mM acetate (FS-acetate). Results are shown as mean±s.e.m. of triplicate of a representative experiment. (c–f) Changes in membrane potential following addition of vehicle or 10 mM acetate to NMC460 (c), HT29 (d) CHOK1 transfected with GPR43 (e) or untransfected (f). Membrane potential was measured using a FLIPR membrane potential assay kit (red) from Molecular Devices. (g) Measurement of Ca2+i mobilization in CHO cells stably expressing GPR43 mediated by 10 mM acetate or vehicle. Data are mean±s.e.m. of duplicates from a representative experiment. (h) Change in membrane potential following addition of vehicle or 10 mM acetate with or without 20 μM BAPTA-AM to NCM460 cells. Membrane potential was measured using a FLIPR membrane potential assay kit (red) from Molecular Devices. Data are mean±s.e.m. of duplicates from a representative experiment. Figure 6: K + efflux or hyperpolarization mediated by acetate induces inflammasome activation in primed human colonic epithelial cells. ( a ) NLPR3 normalized expression with GAPDH was measured in HT29 cells incubated for 2 h with diluted faecal supernatant (FS) or with PBS by real-time PCR. Results are shown as mean±s.e.m. of duplicate of a representative experiment. ( b ) Caspase 1 activity was measured via a fluorometric assay measuring the cleavage of the peptide YVAD-AFC. NMC460 cells were incubated with diluted FS for 4 h followed by 2 h with PBS (FS), incubated with FS for 4 h followed by 2 h in low K + medium (FS-low K + ) or incubated with FS for 4 h followed by 2 h with 10 mM acetate (FS-acetate). Results are shown as mean±s.e.m. of triplicate of a representative experiment. ( c – f ) Changes in membrane potential following addition of vehicle or 10 mM acetate to NMC460 ( c ), HT29 ( d ) CHOK1 transfected with GPR43 ( e ) or untransfected ( f ). Membrane potential was measured using a FLIPR membrane potential assay kit (red) from Molecular Devices. ( g ) Measurement of Ca 2+ i mobilization in CHO cells stably expressing GPR43 mediated by 10 mM acetate or vehicle. Data are mean±s.e.m. of duplicates from a representative experiment. ( h ) Change in membrane potential following addition of vehicle or 10 mM acetate with or without 20 μM BAPTA-AM to NCM460 cells. Membrane potential was measured using a FLIPR membrane potential assay kit (red) from Molecular Devices. Data are mean±s.e.m. of duplicates from a representative experiment. Full size image Fibre affects inflammasome activation via the gut microbiota Fibre not only promotes the release of SCFA through bacterial fermentation but also promotes the growth of beneficial bacteria in the GI tract. We therefore determined to what extent the beneficial effects of fibre in DSS colitis and inflammasome activation was through reshaping gut microbiota composition. A diet deficient in fibre, as well as a high-fibre diet, were fed to mice and then microbiota composition was assessed by culture-independent analyses of amplicons generated across variable regions 1–3 of bacterial 16S ribosomal RNA genes. There were clear and significant differences in gut bacterial composition associated with the three different diets—normal chow, which has an equivalent amount of fibre to that recommended for humans by the DRI, high fibre or zero fibre ( Fig. 7a–c ). Principal coordinate analyses of UniFrac distances of 16S rRNA sequences showed clustering according to diet type, with the most marked change occurring when mice were fed the zero-fibre diet ( Fig. 7a,b ). Relative abundance of bacteria presented at family level ( Fig. 7c ) showed considerably increased levels of Bacteroidiaceae in mice fed a zero-fibre diet compared with normal chow or high-fibre-fed mice. Species notably low or absent from the zero-fibre-fed group were of the family Prevotellaceae , which is consistent with a study that examined microbiota composition of children from Burkina Faso that consumed a high-fibre diet [7] . To identify the bacteria associated with severity of colitis induced by DSS and the production of the inflammasome-related cytokine IL-18, we used Pearson’s correlation ( Fig. 7d ). In addition to Bacteroidetes, Proteobacteria (unclassified, Alcaligenaceae or Helicobacteraceae ), which expanded in Gpr43 −/− mice, and TM7 or Oscillibacter, which expanded in mice fed a no-fibre diet, were also associated with DSS colitis and reduced IL-18 levels ( Fig. 7d ). Of note, Nlrp6 −/− mice were shown to exhibit dysbiosis associated with expansion of TM7 (ref. 17 ), while Proteobacteria (that is, mostly Escherichia coli ) were linked with intestinal inflammation and colitis-associated colorectal cancer [28] . Interestingly, we found that Gpr43 −/− mice were more susceptible to develop colorectal cancer ( Supplementary Fig. 7a–d ), while high-fibre feeding was protective in a GPR43-dependent manner ( Supplementary Fig. 7e ). In contrast, high levels of IL-18 and reduced DSS colitis associated predominantly with other Bacteroidetes (possible some Porphyromonadaceae and Rikenellaceae ) and Firmicutes ( Lachnospiraceae), and these ‘protective’ bacteria were found predominantly in mice fed on a normal chow or high-fibre diet ( Fig. 7d ). 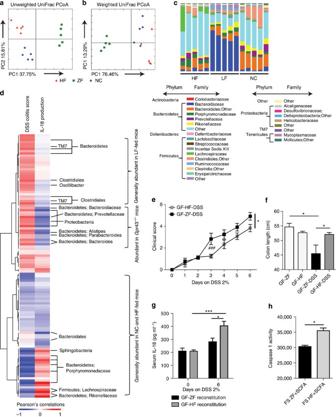Figure 7: High-fibre-fed microbiota is structurally different from zero-fibre-fed microbiota, confers protection in DSS colitis associated and increases inflammasome activation. (a,b) Assessment of structure of microbial communities by unweighted (a) and weighted (b) UniFrac principal coordinate analyses (PCoA) plots are presented for gut bacteria sequenced from mice fed on zero-fibre (ZF), high-fibre (HF) and normal chow diets. (c). Relative abundance of bacteria presented at family level. (d) Pearson’s correlation used to identify the bacteria associated with severity of colitis induced by DSS and the production of the inflammasome-related cytokine IL-18. (e–g) Clinical score (e), colon length (f) and serum IL-18 (g) were determined in GF mice reconstituted with microbiota isolated from HF-fed mice (GF-HF) or from ZF-fed mice (GF-ZF) treated for 6 days on DSS 2 weeks after reconstitution. Mice were fed on normal chow throughout the whole experiment. (h) Caspase 1 activation was measured via a fluorometric assay measuring the cleavage of the peptide YVAD-AFC. NMC460 cells incubated with diluted faecal supernatants from ZF-fed mice (FS ZF) or from HF-fed mice (FS HF) for 4 h and then with 10 mM acetate, 2 mM butyrate and 2 mM propionate for 2 h. The results are shown as mean±s.e.m. with a minimum of five mice per group. With *P<0.05 as a group effect determined by analysis of variance (e),###P<0.001 determined by Tukey’s multiple comparison test (e) and with *P<0.05 and ***P<0.001 as determined byt-test. Figure 7: High-fibre-fed microbiota is structurally different from zero-fibre-fed microbiota, confers protection in DSS colitis associated and increases inflammasome activation. ( a , b ) Assessment of structure of microbial communities by unweighted ( a ) and weighted ( b ) UniFrac principal coordinate analyses (PCoA) plots are presented for gut bacteria sequenced from mice fed on zero-fibre (ZF), high-fibre (HF) and normal chow diets. ( c ). Relative abundance of bacteria presented at family level. ( d ) Pearson’s correlation used to identify the bacteria associated with severity of colitis induced by DSS and the production of the inflammasome-related cytokine IL-18. ( e – g ) Clinical score ( e ), colon length ( f ) and serum IL-18 ( g ) were determined in GF mice reconstituted with microbiota isolated from HF-fed mice (GF-HF) or from ZF-fed mice (GF-ZF) treated for 6 days on DSS 2 weeks after reconstitution. Mice were fed on normal chow throughout the whole experiment. ( h ) Caspase 1 activation was measured via a fluorometric assay measuring the cleavage of the peptide YVAD-AFC. NMC460 cells incubated with diluted faecal supernatants from ZF-fed mice (FS ZF) or from HF-fed mice (FS HF) for 4 h and then with 10 mM acetate, 2 mM butyrate and 2 mM propionate for 2 h. The results are shown as mean±s.e.m. with a minimum of five mice per group. With * P <0.05 as a group effect determined by analysis of variance ( e ), ### P <0.001 determined by Tukey’s multiple comparison test ( e ) and with * P <0.05 and *** P <0.001 as determined by t -test. Full size image We next reconstituted germ-free (GF) mice with the gut microbiota of mice fed on either high- or zero-fibre diets, and subjected them to DSS colitis 2 weeks after reconstitution. These two groups of reconstituted mice were fed the same normal chow diet, so any differences could be attributed to differences in microbiota composition and the effects this has within the gut. Interestingly, we found that GF mice reconstituted with microbiota isolated from high-fibre-fed mice had improved clinical scores ( Fig. 7e ) and increased colon lengths ( Fig. 7f ) when compared with those reconstituted with a zero-fibre-fed microbiota. This protection was correlated with increased IL-18 under DSS conditions but not under basal conditions ( Fig. 7g ). To determine whether microbiota composition could by itself contribute to increased inflammasome activation in epithelium of mice fed a high-fibre diet, NMC460 were primed with either faecal extract isolated from zero- or high-fibre-fed mice and then activated with SCFAs ( Fig. 7h ). Interestingly, the high-fibre microbiota induced significantly more caspase 1 activation compared with zero-fibre, suggesting that changes in bacterial composition participate to fibre-mediated inflammasome activation. Co-housing with WT littermates improves colitis in Gpr43 −/− mice The inflammasome pathway shapes the composition of the gut microbiota, particularly NLRP6 (ref. 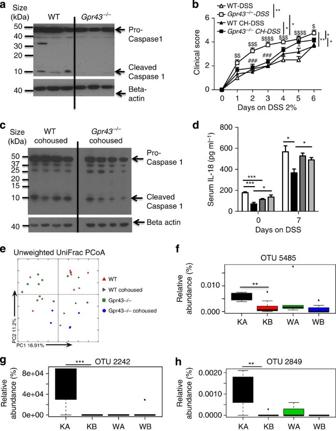Figure 8: Co-housing with WT mice restores colonic epithelium inflammasome activation and improves features of DSS colitis development inGpr43−/−mice. (a,c) Measurement by western blot of cleaved caspase 1 on protein extracted from colonic epithelial cells from WT and fromGpr43−/−mice single-housed (a) or co-housed (c) for 2 weeks before 6 days treatment on DSS 2%. One column represents one mouse. (b,d) Clinical score (b) and IL-18 measured by enzyme-linked immunosorbent assay (d) were assessed in WT (control littermates) single-housed (WT-DSSn=5 mice), in WT co-housed for 2 weeks withGpr43−/−mice (WT CH-DSS,n=6 mice), inGpr43−/−single-housed (Gpr43−/−-DSSn=5 mice) and inGpr43−/−co-housed with WT mice for 2 weeks (Gpr43−/−CH-DSSn=6 mice). Mice were fed on DSS 2% for 6 days. (e–h) Analysis of gut bacterial communities by Observed Species (WT co-housed in orange, WT single-housed in green,Gpr43−/−co-housed in red andGpr43−/−single-housed in blue), unweighted UniFrac principal coordinate analyses (PCoA) plot (e) is presented in single-housed WT (red triangles), in single-housedGpr43−/−mice (green squares), in WT co-housed for 2 weeks withGpr43−/−mice (grey triangles) and inGpr43−/−co-housed for 2 weeks with WT mice (blue circles). Scale bars, 200 μm. (f–h) Increased relative abundance ofPorphyromonadaceaeinGpr43−/−after co-housing. OTUs 5,485 (f), 2,242 (g) and 2,849 (h) of theParabacteroidesgenus, familyPorphyromonadaceae, were found significantly (with respectively ***, **, *** forPvalues 0.0043, 5.5E−4and 0.0010) increased inGpr43−/−mice following co-housing. Representative 16S rRNA sequences were deposited in the EMBL database with sequence accession numbers: HG970160 for OTU5485, HG970161 for OTU2242 and HG970162 for OTU2849. The results are shown as mean±s.e.m. (b,d). With *P<0.05 and **P<0.01 determined by two-way analysis of variance as group effect with$P<0.05,
    P<0.01,
$P<0.001 and
    
P<0.0001 comparing WT versus Gpr43−/−,###P<0.001 comparingGpr43−/−CH versus not CH by Tukey’s multiple analysis and *P<0.05, **P<0.01 and ****P<0.001 determined byt-test. KA: knockout after cohousing; KB: knockout before cohousing; WA: wild-type after cohousing; WB: wild-type before cohousing. 17 ) and NLRP3 (ref. 29 ). Interestingly, deficiency of NLRP6 resulted in an altered, pro-colitogenic gut microflora that was transmissible to co-housed WT mice [17] , as mice are coprophagous. Inflammasome activation is expected in the DSS colitis model, at least in mice on normal chow ( 5
 P <0.01, $$$ P <0.001 and 
    
 P <0.0001 comparing WT versus Gpr43 −/− , ### P <0.001 comparing Gpr 43 −/− CH versus not CH by Tukey’s multiple analysis and * P <0.05, ** P <0.01 and **** P <0.001 determined by t -test. KA: knockout after cohousing; KB: knockout before cohousing; WA: wild-type after cohousing; WB: wild-type before cohousing. Full size image This study emphasizes the importance of dietary fibre for gut homeostasis and outlines precise molecular pathways, whereby fibre impacts on epithelial biology and inflammasome activation. Important in these events is the shaping of the gut microbiome and the fermentation of non-digestible saccharides to high levels of SCFAs, which together are highly effective in activating the inflammasome pathway in colonic epithelium. 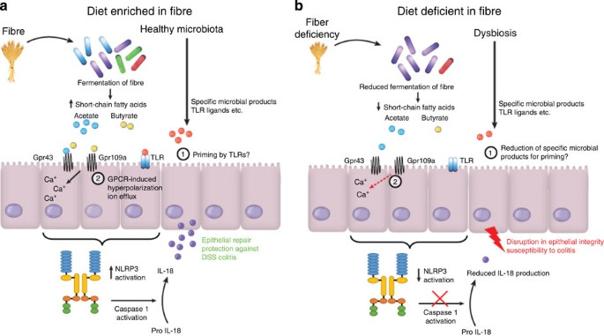Figure 9: A Model of inflammasome activation in gut epithelium, and the role of fibre, gut microbiota, SCFAs and metabolite-sensing GPCRs. (a) Under high-fibre feeding, a contact between the healthy microbiota under injury conditions such as DSS colitis ensures a proper priming of the gut epithelium through products such as TLR ligands. SCFA are highly abundant as a result of fermentation of dietary fibre, which through GPR109A and GPR43 will activate NLRP3 through mechanisms that involve Ca2+i mobilization and membrane hyperpolarization. Activated caspase 1 will cleave IL-18, which will be released promoting epithelial repair and protection from colitis development. (b) On the other hand, dysbiosis linked to consumption of a zero-fibre diet will not promote an optimal priming of the inflammasome and the low level of SCFA and thus decrease signalling of GPR43 and GPR109A will altogether not contribute to proper inflammasome activation. In this situation, IL-18 levels are not properly raised that contribute to exacerbated colitis development. Figure 9 depicts a scheme in which beneficial bacteria expanded through high-fibre feeding as well as their release of SCFA by fermentation of fibre optimally prime and activate the NLRP3 inflammasome in gut epithelium, and thus contribute to gut homeostasis. The priming by bacterial components probably involves a combination of TLR activation, and inflammasome activation by SCFAs occurs through their binding to the metabolite-sensing GPCRs GPR43 and GPR109A. GPR109A has previously been shown to be involved in IL-18 production [30] , and our studies here identify the inflammasome pathway for this increase. Similar to SCFAs, K + efflux activates the inflammasome pathway in primed epithelial cells. SCFAs induce epithelial cell membrane hyperpolarization in a GPR43-dependent manner, suggesting that this mechanism is involved in NLRP3 activation. The release of IL-18 following inflammasome activation contributes to gut homeostasis and protection from colitis. On the other hand, dysbiosis that develops under low-fibre feeding might not effectively prime the inflammasome, and insufficient SCFA signalling through GPCRs might prevent its efficient activation. Figure 9: A Model of inflammasome activation in gut epithelium, and the role of fibre, gut microbiota, SCFAs and metabolite-sensing GPCRs. ( a ) Under high-fibre feeding, a contact between the healthy microbiota under injury conditions such as DSS colitis ensures a proper priming of the gut epithelium through products such as TLR ligands. SCFA are highly abundant as a result of fermentation of dietary fibre, which through GPR109A and GPR43 will activate NLRP3 through mechanisms that involve Ca 2+ i mobilization and membrane hyperpolarization. Activated caspase 1 will cleave IL-18, which will be released promoting epithelial repair and protection from colitis development. ( b ) On the other hand, dysbiosis linked to consumption of a zero-fibre diet will not promote an optimal priming of the inflammasome and the low level of SCFA and thus decrease signalling of GPR43 and GPR109A will altogether not contribute to proper inflammasome activation. In this situation, IL-18 levels are not properly raised that contribute to exacerbated colitis development. Full size image The co-evolution of vertebrates and commensal bacteria over millions of years has resulted in the adaptation of receptors that ‘sense’ bacterial metabolites and facilitate intestinal homeostasis [31] . GPR43 and GPR109A are such receptors, expressed on gut epithelial cells and certain innate immune cells, that respond to SCFAs produced by bacteria in the colon. SCFAs are one of the major products of commensal bacteria, serve as an important source of energy for colonic epithelium, and high production has been identified as a feature of probiotic strains of bacteria [14] . Previous studies by us had identified GPR43 as an important receptor for gut homeostasis, since Gpr43 −/− mice showed increased susceptibility to DSS-induced colitis [12] . GPR43 signals in response to acetate, propionate and to a lesser degree butyrate, and we had speculated that GPR43 was a metabolite-sensing receptor that might somehow facilitate the beneficial effects of dietary fibre for gut health. We also proposed that many diseases associated with western lifestyle may relate to insufficient intake of dietary fibre [8] . We found here that deficiency of dietary fibre did indeed compromise, whereas high-fibre diet promoted gut homeostasis. The importance of GPR43 and GPR109A for these effects was clearly evident through analysis of histological scores, colon length and clinical scores in the DSS model. We do not exclude a role for other metabolite-sensing GPCRs, of which there are a growing number [4] ; however, an acetate binding receptor is likely one of the most important given the findings by Fukuda et al. [14] who identified acetate as important for gut barrier function. The inflammasome pathway is critical for epithelial integrity by ensuring repair and cell survival under stress conditions. However, upstream mechanisms of inflammasome activation in epithelium have been poorly characterized. As in macrophages, we found that hyperpolarization mediated by K + efflux efficiently promoted NLRP3 inflammasome activation in primed epithelial cells. K + efflux is a mechanism that can develop under stress condition to protect cell integrity. Endoplasmic reticulum stress in epithelium has been associated with inflammatory bowel disease and in vitro exposure of colonic epithelial cells to endoplasmic reticulum stress causes rapid K + efflux [32] . Such a mechanism may contribute to epithelial inflammasome activation in colitis. Similar to K + efflux, we found that acetate mediated hyperpolarization through GPR43 and activated the inflammasome in colonic epithelial cells. As described for neutrophils [12] , [33] , acetate induced an increase in intracellular Ca 2+ in colonic epithelial cells, which is in accordance with other reports showing enteroendocrine cells expressing GPR43 mobilize Ca 2+ when stimulated with agonist [34] . An increase of intracellular Ca 2+ has been shown to promote K + efflux in HT29 cells, suggesting that the hyperpolarizing effects of acetate might be due indirectly to a rise in intracellular Ca 2+ (ref. 35 ). A recent study found that Ca 2+ mobilization is a common, proximal step in activation of the NLRP3 inflammasome [36] . These authors speculated that the many mechanisms for mobilizing Ca 2+ , including GPCR activation, may be relevant for NLRP3 activation [36] . Our present finding support this, as addition of a Ca 2+ chelator to epithelial cells blocked the hyperpolarizing effects of acetate. Similar to GPR43, activation of other SCFA receptors such as GPR41 and GPR109A induces intracellular Ca 2+ mobilization in neutrophils [33] , [37] , and presumably the same occurs in colonic epithelial cells, resulting in inflammasome activation and gut homeostasis. This might explain why high-fibre feeding still had a beneficial role in Gpr43 −/− and Gpr109A −/− mice. We found that direct contact of epithelial cells with faecal extract was able to prime the NLRP3 inflammasome, and then SCFA could activate this pathway. Priming consists notably of increased expression of pro-IL-18 (ref. 38 ). Interestingly, activation was increased when cells were primed with a healthy microbiota, emphasizing the likely contribution of bacterial products to both signal 1 and signal 2 (that is, SCFAs). Using Pearson’s correlation, we identified bacterial strains that positively correlated with IL-18 release in vivo , signifying increased inflammasome activation, and these also correlated negatively with colitis severity. Candidates such as Lachnospiraceae , a producer of butyrate [39] , and Rikinellaceae and Porphyromonadaceae, both producers of acetate and propionate [40] , and Sphingobacteria were identified. Mechanisms whereby these species might directly contribute to signal 1 in epithelial cells are unclear but may involve TLR signalling, as these bacterial species have been linked to Myd88 (ref. 41 ), Irak [42] , TLR5 (ref. 43 ) and TLR4 (ref. 44 ). Signalling through GPR43 may not always result in Ca 2+ mobilization and inflammasome activation. Another important function of SCFAs in the colon is regulation of inducible Treg numbers [45] , [46] , [47] , which is another mechanism that contributes to gut homeostasis. There are other pathways besides inflammasome activation whereby GPR43 signalling may affect cell functions, including β-arrestin2 signalling, an alternative pathway activated by many metabolite-sensing GPCRs including GPR43. Circumstances whereby GPR43 stimulation by its agonists results in β-arrestin2 versus conventional G-protein signalling (and Ca 2+ mobilization) are still unclear. However, regardless of the precise signalling pathways, GPR43 promotes numerous events for proper gut and immune homeostasis, including epithelial integrity via inflammasome activation, anti-inflammatory effects (probably through β-arrestin2 activation) and promotion of inducible Treg numbers through histone deacetylase inhibition. The detrimental effects of low-fibre intake (or deficiency of GPR43) we observed in mouse models of colitis may have parallels with human populations that consume inadequate amounts of fibre. Certainly, epidemiological studies on nutrition and human disease would support this [9] , [11] . Further studies in humans will be required to determine the precise relevance of dietary fibre, versus other variables such as high-fat intake, for human diseases. Insight into molecular pathways that connect diet to intestinal homeostasis, exemplified here, may herald new approaches based on diet, prebiotics and probiotics to prevent or treat a range of human diseases. The connection of the inflammasome pathway in epithelium to dietary metabolites and metabolite-sensing GPCRs should allow both natural and pharmaceutical approaches to the treatment or prevention of human disease. Reagents and diets DSS was purchased from MP Bioscience (Mw: 35–43 kDa). Coating and detection anti IL-18 antibodies used for enzyme-linked immunosorbent assay were obtained from MBL and AOM from Sigma-Aldrich. Rabbit anti-mouse caspase 1 was obtained from Santa Cruz Biotechnology, rat anti-mouse IL-18 from MBL and mouse anti-β-actin from Cell Signaling. Goat horseradish peroxidase-conjugated anti-mouse, anti-rabbit, anti-rat and mouse anti-goat antibodies were obtained from Jackson ImmunoResearch Laboratories. Primer sequences used for real-time PCR were NLRP3 forward 5′-CACCTGTTGTGCAATCTGAAG-3′, reverse 5′-GCAAGATCCTGACAACATGC-3′ and GAPDH forward 5′-GCCCAATACGACCAAATCC-3′ and reverse 5′-AGCCACATCGCTCAGACAC-3′. The different diets, high fibre (SF11-029), zero fibre (SF11-028), low fibre (SF13-055), resistant starch (SF11-025) and normal chow (AIN93G) were all purchased from Speciality Feeds, Glenn Forest, Australia. Animals and models All experimental procedures involving mice were carried out according to protocols approved by the Animal Ethics Committees of Monash and Yale Universties. Gpr43 −/− mice were obtained from Deltagen and crossed ~13 generations to a C57Bl/6 background, control littermates were used as WT for the co-housing experiments. Gpr109A −/− mice on a C57Bl/6 background have been described [48] and were kindly provided by Professor Stephan Offermans, Max Plank institute, Bad Nauheim. Nlrp 3 −/− mice were kindly provided by Professor Mansell, Monash University. Nlrp 6 −/− mice were housed in Yale University and were on a C57Bl/6 background. Throughout the whole study, mice were randomly chosen to be fed on different diets and were given diets for at least 7 days before starting DSS, at a minimum age of 6 weeks. DSS colitis : mice from 7 to 9 weeks were fed as specified in the text, and DSS was added to the drinking water (percentage indicated in each figure) for 6 days and were monitored daily. A minimum of n =5 mice per group were used to reach significance as published before [12] and were scored blind. The clinical score ranging from 1 to 8 was assessed as follows: 0, no sign of disease; 1, positive hemoccult normal faeces; 2, positive hemoccult soft faeces; 3, positive hemoccult pasty faeces; 4, positive hemoccult liquid faeces; 5, moderate rectal bleeding; 6, severe rectal bleeding; 7, haemorrhagia and 8, death. Colon histology scoring was done blindly on paraffin-embedded colon section stained with haematoxylin and eosin and ranged from 0 to 6 by adding the tissue damage scoring (0, no mucosal damage; 1, lymphoepithelial lesions; 2, surface mucosal erosion and 3, extensive mucosal damage, extension into deeper structure) to the inflammatory cell infiltration scoring (0, occasional cell infiltrate; 1, increased number of infiltrating cells; 2, confluency of inflammatory cells extending to the submucosa and 3, transmural extension of the inflammatory cells). Colon length was measured after 6 days of treatment with DSS. Under basal conditions, mice losing >15% body weight were killed and excluded from the study. Acetate treatment in drinking water An amount of 100, 200 or 300 mM sodium acetate (Sigma) was given in drinking water (fresh solutions three times a week) for 3 weeks before DSS treatment. The mice remained on acetate during the DSS treatment. SCFAs measurements Serum and faecal acetate measurements were made by nuclear magnetic resonance at the Bio21 at Melbourne University. Serum was isolated from blood harvested by heart puncture, faeces were sterilely harvested and frozen on dry ice immediately after harvest. Serum measurements were done on mice fed for 7 and 14 days on diets and faecal measurement on mice fed for 14 days on diets. Cleaved caspase 1 and IL-18 western blots Western blots were performed on intestinal epithelial cell isolated following a protocol adapted from a method previously described [17] . Briefly, colons were cut in small pieces and incubated in a solution of Hank's balanced salt solution with 5 mM EDTA and 1 mM dithiothreitol for 40 min at 37 °C under agitation, samples were then filtered through 100 μM porous membrane and centrifugated for 5 min at 1,500 r.p.m. The centrifugated pellet represents the intestinal epithelial cells. Reconstitution of GF mice with microbiota Colonic and caecal concents from high- versus zero-fibre-fed mice were resuspended in sterile-cold PBS at a concentration of 100 mg ml −1 and then vortexed. The suspension was filtered through 70 μm filters and 5-week-old female C57Bl/6 GF mice, housed in sterile isolators, were gavaged with 200 μl of this solution. Two weeks after reconstitution, mice were treated (or not) with DSS. Bone marrow chimaeras Recipient 6-week-old mice were irradiated with two doses of 4.75 Gy 6 h apart. They were reconstituted the day after by intravenous injection of 5 million bone marrow cells isolated from 6-week-old mice. Different diets were started 8 weeks after irradiation and the DSS treatment 1 week after the diet started. Study of membrane potential changes Cells used throughout our studies were confirmed negative for mycoplasma using MycoAlert mycoplasma detection kit (Lonza). Cells were seeded at 40,000 or 80,000 cells per well for CHOK1 and HT29 cells, respectively, into clear 96-well tissue culture plates. Cells were incubated overnight and were washed once with PBS the following day. An amount 90 μl HBSS (145 mM NaCl, 22 mM HEPES, 0.34 mM Na 2 HPO 4 , 4.2 mM NaHCO 3 , 0.44 mM KH 2 PO 4 , 0.41 mM MgSO 4 , 0.49 mM MgCl 2 , 1.3 mM CaCl 2 and 5.6 mM glucose, pH 7.4) were added to each well followed by 90 μl membrane potential assay kit dye (red; Molecular Devices, Sunnyvale, CA) reconstituted in assay buffer supplied with the kit, which was HBSS as described previously, with 5.33 mM KCl. Thus, the final concentration of KCl in the assay was 2.67 mM. Cells were incubated at 37 °C for 45 min before the addition of 20 μl acetate or vehicle. Fluorescence was measured using a FlexStation 3 microplate reader (Molecular Devices) with an excitation at 530 nm and emission at 565 nm. Baseline readings were taken for 30 s before acetate or vehicle addition. Changes in fluorescence following acetate or vehicle addition were measured for 800 s and expressed as relative fluorescent units following baseline subtraction. A reduction in fluorescence intensity represents hyperpolarization of the cell membrane owing to the assay dye following the positively charged ions out of the cell, whereas an increase in intensity reflects depolarization. Concerning the Ca 2+ chelator experiment, cells were seeded at 50,000 cells per well into clear 96-well tissue culture plates and incubated for 48 h. On the day of the assay, cells were washed once with PBS. A quantity of 90 μl low potassium HBSS (145 mM NaCl, 22 mM HEPES, 0.34 mM Na 2 HPO 4 , 4.2 mM NaHCO 3 , 0.44 mM KH 2 PO 4 , 0.41 mM MgSO 4 , 0.49 mM MgCl 2 , 1.3 mM CaCl 2 and 5.6 mM glucose, pH 7.4) were added to each well followed by 90 μl membrane potential assay kit dye (red; Molecular Devices, Sunnyvale, CA) reconstituted in assay buffer supplied with the kit, which was HBSS as described previously, with 5.33 mM KCl. Thus, the final concentration of KCl in the assay was 2.67 mM. Cells were incubated at 37 °C for 15 min before the addition of 4 μl vehicle or 1 mM BAPTA-AM for a final concentration of 20 μM. Cells were incubated for a further 30 min before the addition of 20 μl acetate at a final concentration of 10 mM or vehicle. Fluorescence was measured using a FlexStation 3 microplate reader (Molecular Devices) with an excitation at 530 nm and emission at 565 nm. Baseline readings were taken for 30 s before acetate or vehicle addition. Changes in fluorescence following acetate or vehicle addition were measured for 800 s and expressed as RFUs following baseline subtraction. The response of the cells to vehicle was subtracted from the response to acetate. A reduction in fluorescence intensity represents hyperpolarization of the cell membrane owing to the assay dye following the positively charged ions out of the cell, whereas an increase in intensity reflects depolarization. Caspase 1 activity One million NMC460 cells per well were seeded in 12-well plate and differentiated in F12:Ham medium complemented with 10% heat-inactivated fetal bovine serum for a week. Faecal pellets from zero-fibre-fed mice or high-fibre-fed mice were collected and homogenized in sterile PBS at a concentration of 100 mg ml −1 . Resulting supernatant was then collected after filtering through a 70-μM cell strainer and then diluted 1,000 times in PBS. Cells were stimulated with 500 μl of supernatant for 4 h and then either stimulated with PBS for 2 h, low K+ medium (made in Milli-Q water contained (in mM) NaCl 145, HEPES 22, Na 2 HPO 4 0.338, NaHCO 3 4.17, KCl 5.33, KH2PO 4 0.441, MgSO 4 0.407, MgCl 2 0.493, CaCl 2 1.26 and glucose 5.56 (pH 7.4, osmolarity 315±5)), 10 mM acetate (Sigma-Aldrich, St Louis, USA) or combination of 10 mM acetate and 2 mM butyrate (Sigma-Aldrich) and 2 mM propionate (Sigma-Aldrich). Caspase 1 activity was measured using the caspase 1 fluorometric assay kit 3484 (BioVision, San Francisco, USA) according to manufacturer’s instructions. Bacteria DNA sequencing and bioinformatics The structure of microbial communities was assessed using both the presence or absence information (unweighted Unifrac) and relative abundance data (weighted Unifrac). Faecal samples were stored at −80 °C before use. DNA was purified using QIAamp DNA stool mini kit (Qiagen). DNA samples were amplified using V2-V3 region primers targeting bacterial 16s rRNA gene and sequenced using Roche 454 sequencer. Initial bioinformatics analysis was carried out using the QIIME 1.5.0 software ( http://qiime.org/index.html ) and used default parameter settings. We performed single even-depth rarefaction analysis. Taxonomies were assigned with Ribosomal Database Project. Difference of bacteria taxa populations among the mice groups were statistically evaluated by analysis of variance with P =0.05 as the statistical significance cutoff. Associations between DSS score/IL-18 production and individual taxa proportions were assessed by Pearson’s correlation coefficient. Representative 16S rRNA sequences were deposited in the EMBL database with the following sequence accession numbers: HG970160 for OTU5485, HG970161 for OTU2242 and HG970162 for OTU2849. Inflammation-induced colon cancer Mice were given a single intraperitoneal injection (10 mg per kg body weight) of AOM. Mice were treated with 2.5% DSS for 5 days, followed by 16 days of regular drinking water. This cycle was repeated twice and mice were killed 12 weeks post-AOM injection or when the animals were moribund. How to cite this article: Macia, L. et al. Metabolite-sensing receptors GPR43 and GPR109A facilitate dietary fibre-induced gut homeostasis through regulation of the inflammasome. Nat. Commun. 6:6734 doi: 10.1038/ncomms7734 (2015).